Interaction of independent single photons based on integrated nonlinear optics The parametric interaction of light beams in nonlinear materials is usually thought to be too weak to be observed when the fields involved are at the single-photon level. However, such single-photon level nonlinearity is not only fundamentally fascinating but holds great potential for emerging technologies and applications involving heralding entanglement at a distance. Here we use a high-efficiency waveguide to demonstrate the sum-frequency generation between a single photon and a single-photon level coherent state. The use of an integrated, solid state, room temperature device and telecom wavelengths makes this type of system directly applicable to future quantum communication technologies such as device-independent quantum key distribution. Photons are ideal carriers of quantum information, as they can be easily created and can travel long distances without being affected by decoherence. For this reason, they are well suited for quantum communication [1] . However, the interaction between single photons is negligible under most circumstances. Realizing such an interaction is not only fundamentally fascinating but holds great potential for emerging technologies. It has recently been shown that even weak optical nonlinearities between single photons can be used to perform important quantum communication tasks more efficiently than methods based on linear optics [2] , which have fundamental limitations [3] . Nonlinear optical effects at single-photon levels in atomic media have been studied [4] , [5] and demonstrated [6] , [7] , [8] , [9] , but these are neither flexible nor compatible with quantum communication, as they impose restrictions on photons’ wavelengths and bandwidths. Here we use a high-efficiency nonlinear waveguide (WG) [10] , [11] to observe the sum-frequency generation (SFG) between a single photon and a single-photon level coherent state from two independent sources. The potential of parametric interactions used for quantum information processing has been demonstrated in a variety of interesting experiments [12] , [13] , [14] . Although these interactions have been shown to preserve coherence [15] , [16] , [17] , they are generally performed using strong fields [18] , [19] , [20] . It is only recently that parametric effects such as cross-phase modulation [21] , [22] and spontaneous downconversion [23] , [24] have been observed with a single-photon level pump. We take the next step and realize a photon–photon interaction, which can enable some fascinating experiments. For example, Fig. 1 shows how the SFG of two photons γ 2 and γ 3 from independent spontaneous parametric down conversion (SPDC) sources can herald the presence of two distant photons γ 1 and γ 4 , as proposed in ref. 2 . If the photon pairs are initially entangled using time-bin encoding, the detection of the photon γ 5 on a basis that erases the ‘which path’ information about its creation time projects the pair γ 1 γ 4 in an entangled state. If we compare this approach for the heralded creation of entangled pairs with the linear optics scheme presented in ref. 25 (which is shown to be optimal with respect to the number of photon pairs needed), to obtain a generated state with fidelity F ≥0.9, and assuming an overall detection and coupling efficiency of η =0.6, our nonlinear optical proposal represents a competitive alternative as soon as the efficiency [2] of the SFG is 10 −8 . Such efficiencies of 10 −8 are, however, extremely challenging to achieve in common nonlinear crystals. 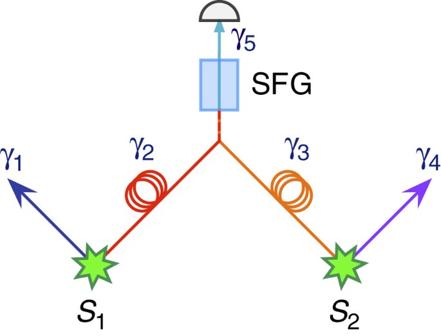Figure 1: Concept. The SFG of photons from separate sources. A photon from each of two pair sourcesS1andS2is sent over a distance to a nonlinear WG. This WG performs the sum-frequency generation (SFG) of photons γ2and γ3and outputs a photon γ5. Detecting this photon heralds the distant presence of photons γ1and γ2. Critically, the SFG process will work only for γ2and γ3and not for two photons coming from the same source. This feature would allow for faithful entanglement swapping, which is otherwise impossible to perform with two probabilistic pair sources and linear optics. Figure 1: Concept. The SFG of photons from separate sources. A photon from each of two pair sources S 1 and S 2 is sent over a distance to a nonlinear WG. This WG performs the sum-frequency generation (SFG) of photons γ 2 and γ 3 and outputs a photon γ 5 . Detecting this photon heralds the distant presence of photons γ 1 and γ 2 . Critically, the SFG process will work only for γ 2 and γ 3 and not for two photons coming from the same source. This feature would allow for faithful entanglement swapping, which is otherwise impossible to perform with two probabilistic pair sources and linear optics. Full size image In our experiment, we increase the interaction cross-section by strongly confining the photons, both spatially and temporally, over a long interaction length. The spatial confinement is achieved with a state-of-the-art nonlinear WG [10] , [11] , whereas the temporal confinement is obtained by using pulsed sources [26] . The efficiency of the process is proportional to the square of the WG length L 2 and inversely proportional to the duration of the input photons. L is limited by the group velocity dispersion between the input photons and the unconverted photon [2] . We maximize the SFG efficiency by matching the spectrotemporal characteristics of the single photons with the phase-matching constraints of the WG. A 4-cm WG and 10-ps photon satisfy these conditions. The use of an integrated, room temperature device and telecom wavelengths makes this approach to photon–photon interaction well adapted to long-distance quantum communication, moving quantum nonlinear optics one step further towards complex quantum networks and future applications such as device-independent quantum key distribution. Sources A schematic of the experimental set-up is shown in Fig. 2 . A 532-nm mode-locked laser produces pulses that pump two distinct sources. The first source produces pairs of photons by spontaneous parametric downconversion at 807 and 1,560 nm (SPDC source). Further details can be found in ref. 26 . The second source produces weak coherent state pulses at 1,551 nm by difference frequency generation (DFG) source. The process is stimulated by a 810-nm continuous wave seed laser. The average number of photons in the coherent state pulse can be adjusted by changing the seed and pump powers. All photons are coupled into single-mode fibres. 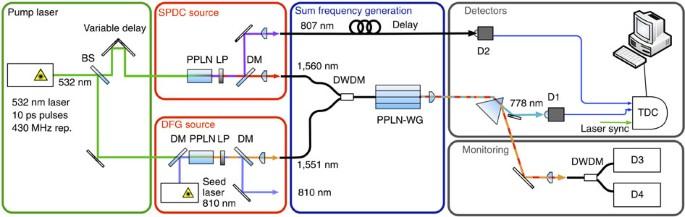Figure 2: Experimental set-up. A mode-locked laser that generates 10 ps pulses at 532 nm with a repetition rate of 430 MHz is used to pump the two sources. The SPDC source consists of a periodically poled lithium niobate (PPLN) crystal set to produce pairs of photons at 807 and 1,560 nm. These are deterministically separated by a dichroic mirror (DM) and collected into optical fibres. The remaining pump light is removed with a long pass filter (LP). The DFG source consists of a similar PPLN crystal seeded by a continuous wave laser at 810 nm producing coherent state pulses at 1,551 nm by DFG. These pulses are combined into the same fibre via a 200-GHz three-port dense wavelength divsion multiplexer (DWDM; ACPhotonics) and directed to the PPLN waveguide (WG). The PPLN-WG is 4.5 cm long and has a SHG efficiency of 41% W−1cm−2at 1,556 nm. The upconverted light is separated from the remaining telecom light via a prism, and sent to D1, a free space Si detector. The remaining unconverted telecom light is demultiplexed by another DWDM and sent to detectors D3 and D4, two free running InGaAs detectors. D3 and D4 are used for monitoring the coupling stability during the experiment and for optimizing the transmission of the input fields through the WG by optimising their polarization. We record threefold coincidences between detectors D1, D2 and the laser clock signal using a time-to-digital converter (QuTools). Figure 2: Experimental set-up. A mode-locked laser that generates 10 ps pulses at 532 nm with a repetition rate of 430 MHz is used to pump the two sources. The SPDC source consists of a periodically poled lithium niobate (PPLN) crystal set to produce pairs of photons at 807 and 1,560 nm. These are deterministically separated by a dichroic mirror (DM) and collected into optical fibres. The remaining pump light is removed with a long pass filter (LP). The DFG source consists of a similar PPLN crystal seeded by a continuous wave laser at 810 nm producing coherent state pulses at 1,551 nm by DFG. These pulses are combined into the same fibre via a 200-GHz three-port dense wavelength divsion multiplexer (DWDM; ACPhotonics) and directed to the PPLN waveguide (WG). The PPLN-WG is 4.5 cm long and has a SHG efficiency of 41% W −1 cm −2 at 1,556 nm. The upconverted light is separated from the remaining telecom light via a prism, and sent to D1, a free space Si detector. The remaining unconverted telecom light is demultiplexed by another DWDM and sent to detectors D3 and D4, two free running InGaAs detectors. D3 and D4 are used for monitoring the coupling stability during the experiment and for optimizing the transmission of the input fields through the WG by optimising their polarization. We record threefold coincidences between detectors D1, D2 and the laser clock signal using a time-to-digital converter (QuTools). Full size image The telecom photons generated by the SPDC source are combined with the coherent state pulses from the DFG source using a dense wavelength division multiplexer (DWDM). We verified the single-photon nature of the SPDC source by measuring the conditional second-order correlation function of the telecom photon after the DWDM to be g (2) (0)=0.03. SFG device The photons are then sent to a fibre pigtailed reverse proton exchange type 0 periodically poled lithium niobate WG, 4.5 cm long [10] . This WG produces SFG of the input fields according to the phase-matching conditions shown in Fig. 3 . 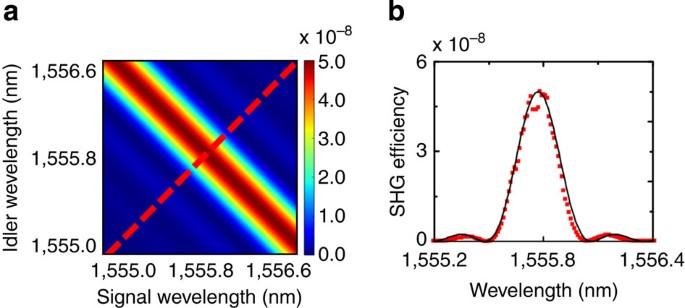Figure 3: WG efficiency. (a) Calculation of the WG efficiency taking into account the quasi-phase-matching conditions. The red-dashed line represents points corresponding to SHG. (b) Measured values for the efficiency of SHG (red points) compared with the theoretical prediction (solid line), showing an almost ideal phase-matching of the PPLN-WG. Figure 3: WG efficiency. ( a ) Calculation of the WG efficiency taking into account the quasi-phase-matching conditions. The red-dashed line represents points corresponding to SHG. ( b ) Measured values for the efficiency of SHG (red points) compared with the theoretical prediction (solid line), showing an almost ideal phase-matching of the PPLN-WG. Full size image The overall system efficiency for second harmonic generation (SHG) is measured to be 41% W −1 cm −2 at 1,556 nm, and is used to estimate the SFG efficiency as described in the Methods. In addition to high efficiency, the WG exhibits almost ideal phase matching, as can be seen from Fig. 3b , as well as a high coupling of the fibre to the WG of 70%. Measurement results To verify the signature of our photon–photon interaction, we record threefold coincidences between detectors D1 and D2 (both Si detectors) and the laser clock signal. When an upconverted photon is detected at D1 (3.5 Hz dark counts, 62% detection efficiency at 780 nm), an electric signal is sent to D2 (probability of dark count per gate 10 −3 , detection efficiency 40% at 810 nm) [27] opening a 10-ns-detection window. Conditioning the upconversion events on the laser clock signal helps to reduce the noise. We ensure that the photons arrive at the same time inside the WG by moving a motorized delay. 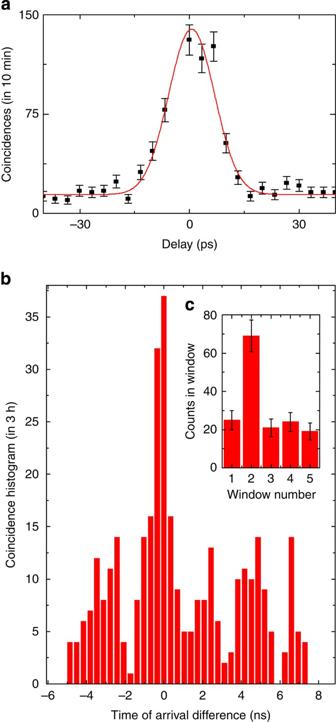Figure 4: Temporal delay and coincidence measurement. (a) Temporal overlap of input signals at the WG measured by introducing a delay between the photons’ arrival times. The Gaussian fit (solid line) gives a FWHM 14.8 ps, which corresponds to a convolution of two pulses of 10 ps from our laser. The spectra of the SPDC and of the DFG are, respectively, 1.2 nm and 0.8 nm, corresponding to 6.76 ps and 10.03 ps, respectively. This indicates that to within the resolution of our measurement, our photons are close to being single mode. (b) Coincidence histogram between D1 and D2 showing strict time correlation between the heralding upconverted photon and the 807 nm photon. The spread of the coincidence peak is mainly dominated by detector jitter. Side peaks are due to the periodicity of the laser. (c) Bar chart histogram is obtained by integrating the two central bins of each peak. Error bars, 1 s.d. Figure 4a shows the upconverted signal as a function of the delay between the photons. When performing this temporal alignment, the mean number of photons in the coherent state was increased to 25 per pulse. Each point of Fig. 4a corresponds to the number of threefold coincidences between D1, D2 and the laser clock that occur over 10 min. The full width at half maximum (FWHM) of the graph seen in Fig. 4 is 14.8 ps, which corresponds to the convolution of two 10 ps pulses from the pump laser. From the spectra of the photons that are 1.2 nm for the SPDC and 0.8 nm for the DFG, we can deduce their coherence times, respectively, 6.76 and 10.03 ps. This is a good indication that our photons are close to being pure. Figure 4: Temporal delay and coincidence measurement. ( a ) Temporal overlap of input signals at the WG measured by introducing a delay between the photons’ arrival times. The Gaussian fit (solid line) gives a FWHM 14.8 ps, which corresponds to a convolution of two pulses of 10 ps from our laser. The spectra of the SPDC and of the DFG are, respectively, 1.2 nm and 0.8 nm, corresponding to 6.76 ps and 10.03 ps, respectively. This indicates that to within the resolution of our measurement, our photons are close to being single mode. ( b ) Coincidence histogram between D1 and D2 showing strict time correlation between the heralding upconverted photon and the 807 nm photon. The spread of the coincidence peak is mainly dominated by detector jitter. Side peaks are due to the periodicity of the laser. ( c ) Bar chart histogram is obtained by integrating the two central bins of each peak. Error bars, 1 s.d. Full size image Once the SPDC and DFG sources have been characterized, we set the temporal delay to zero and measure the performance of the nonlinear interaction. For this measurement, the coherent state had a mean number of 1.7 photons per pulse inside the WG. A histogram of arrival time differences is shown in Fig. 4b (each bin corresponds to 0.32 ns). The main peak is the signature of photon–photon conversion. It is also possible to see side peaks, which correspond to a dark count at D1 owing to intrinsic noise of the detector followed by a detection of a photon at D2 (see Methods). The periodicity of these side peaks corresponds to the period of the pump laser. To more clearly see the signal-to-noise characteristics of the experiment, we integrate over the events in the two central bins for each peak. This is shown in Fig. 4c , where a peak with a signal-to-noise of 2 can be seen. The coincidence rate between D1 and D2 was 25±5 counts per hour. To determine the efficiency of the SFG, we can use this rate along with other independently measured parameters from our set-up. We estimate the overall efficiency of the process at the single-photon level to be η SFG =(1.5±0.3) × 10 −8 . Alternatively, using the measurement of SHG efficiency, the calculation of the SFG efficiency shown in Fig. 3 and accounting for the bandwidth of the interacting beams, we estimated the efficiency to be 1.56 × 10 −8 , which agrees well with the value estimated from the measured data. We highlight that this is the overall conversion efficiency, which includes the effects of coupling into the WG, internal losses and losses through the set-up up to D1. Correcting for all of these losses, we obtain the intrinsic device efficiency of (2.6±0.5) × 10 −8 . We have demonstrated the nonlinear interaction between a single photon and a single-photon level coherent state. Such single-photon level parametric interactions open new perspectives for emerging quantum technologies. At the level of efficiency (1.5 × 10 −8 ) demonstrated here, the technique is already competitive with linear optics protocols [25] , [28] , [29] , and offers new possibilities such as heralding entanglement at a distance [2] . This approach also opens the way towards device-independent quantum key distribution [30] . Unlike previously proposed linear optics schemes, there is significant scope for improvements as higher nonlinearities are realised. Work in this field is advancing rapidly, using materials with higher nonlinear coefficients [31] as well as methods for tighter field confinement [32] . The use of an integrated, solid state, room temperature device and a flexible choice of wavelengths will further aid the applicability of this type of system in future quantum communication technologies and beyond. Evaluation of the number of photons in the coherent state To evaluate the number of photons per pulse in the coherent state, we measure the average power P α at the output of the DWDM. The average number of photons per pulse at this point is where f is the laser repetition rate of 430 MHz. To have the number of photons inside the WG, we multiply by the overall transmission of the set-up from the DWDM to the interior of the WG, including the coupling of the pigtail inside the WG of 70%. The overall transmission is 64%. Noise characterization Understanding the origin of the side peaks present in the graph of Fig. 5 is crucial. To do this, we blocked the telecom photon coming from the SPDC source but not the coherent state from the DFG source, and recorded threefold coincidences between D1, D2 and the laser clock. The scaling of such noise in detector D2 as a function of the average power in the coherent state can be seen in Fig. 5 . Each point in the graph corresponds to a coincidence histogram integrated over 20 min. The quadratic behaviour of this noise suggests a possible contribution of SHG from 1,551-nm pulses to these side peaks. 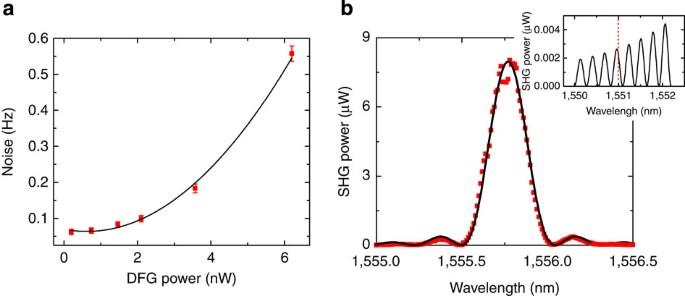Figure 5: Noise in D2 and SHG. (a) Quadratic behaviour of noise in detector D2 as a function of DFG source power. (b) The SHG spectrum. Solid line indicates fit of the data with a sinc2function. (Inset: zoom of fit) Dashed red line shows the predicted intensity of SHG at 1,551 nm. Error bars, 1 s.d. Figure 5: Noise in D2 and SHG. ( a ) Quadratic behaviour of noise in detector D2 as a function of DFG source power. ( b ) The SHG spectrum. Solid line indicates fit of the data with a sinc 2 function. (Inset: zoom of fit) Dashed red line shows the predicted intensity of SHG at 1,551 nm. Error bars, 1 s.d. Full size image To evaluate this, we estimate the effective SHG efficiency from the second harmonic spectrum seen in Fig. 4b . The peak value of such spectrum corresponds to a measured efficiency of 41% W −1 cm −2 . From a fit of such a spectrum, we conclude that the effective SHG efficiency for 1,551 nm is η SHG (1,551) =2.35 10 −4 × 41% W −1 cm −2 . Taking into account this effective efficiency, we can estimate the expected rates at detector D1 due to SHG of the coherent state pulses. These rates are simply where μ is the coupling efficiency of the coherent state into the optical fibre, which was measured to be 76% and L is the length of the WG. The result of this estimation compared with the actual measured values can be seen in Table 1 . Table 1 Noise in D1 as a function of the coherent state size. Full size table From such an analysis, we can conclude that the SHG contribution to the noise at the single-photon level can be neglected. The side peaks are then dominated by coincidence between a dark count at D1 and a detection at D2. This confirms that a detection of an upconverted photon does not come from conversion of two photons from the same DFG pulse. SFG efficiency measurement Using the data shown in Fig. 5 , we can extract the rate of coincidences between D1 and D2, R SFG . By combining these with other numbers from the set-up, independently characterised, we can then extract the overall SFG efficiency from a single-photon measurement. The numbers used to obtain this efficiency can be seen in Table 2 . Table 2 Key parameters of the set-up. Full size table The SFG efficiency is then given by where β is the product of all the quantities in Table 2 times the laser repetition rate of 430 MHz. From the experimental data, we obtained R SFG =25±5 counts per hour, yielding an overall efficiency of η SFG = (1.5 ± 0.3) × 10 −8 . SFG efficiency estimation It is natural to ask whether the value found for the SFG efficiency agrees with the value for the efficiency of the SHG, measured classically, shown in Fig. 3 . To do that, we modelled the phase-matching conditions of the WG using the appropriate Sellmeier equations [33] . The peak value of the SHG efficiency, corresponding to a wavelength of 1,556 nm, is 41% W −1 cm −2 . Given an efficiency measured at the classical level η , we can obtain the corresponding value at the single-photon level using the equation [2] where for our system, L =4.5 cm, ≥296 GHz cm and tbp= 0.66. To give an example, the peak level for the SHG efficiency then reads , which is of the same order of magnitude of the SFG efficiency obtained experimentally. This estimation, however, did not take into account the bandwidth of the interacting fields. To take this into consideration, we use the matrix shown in Fig. 3 to obtain , the efficiency as a function of the wavelengths of the input fields. We then integrate over the spectra of the interacting beams, normalized to the area, denoted by p s ( λ s ) and p i ( λ i ). The total effective efficiency reads which is in agreement with the value found from the measured data. Accession codes : The complete consensus mt genome sequences have been deposited to NCBI GenBank under Accession numbers KC553980 – KC554018 . How to cite this article: Guerreiro, T. et al . Interaction of independent single photons based on integrated nonlinear optics. Nat. Commun. 4:2324 doi: 10.1038/ncomms3324 (2013).